Room temperature magnetic materials from nanostructured diblock copolymers Nanostructured magnetic materials are important for many advanced applications. Consequently, new methods for their fabrication are critical. However, coupling self-assembly to the generation of magnetic materials in a simple, straight-forward manner has remained elusive. Although several approaches have been considered, most have multiple processing steps, thus diminishing their use of self-assembly to influence magnetic properties. Here we develop novel block copolymers that are preprogrammed with the necessary chemical information to microphase separate and deliver room temperature ferromagnetic properties following a simple heat treatment. The importance of the nanostructured confinement is demonstrated by comparison with the parent homopolymer, which provides only paramagnetic materials, even though it is chemically identical and has a higher loading of the magnetic precursor. In addition to the room temperature ferromagnetic properties originating from the block copolymer, the in situ generation densely functionalizes the surface of the magnetic elements, rendering them oxidatively stable. Magnetic materials remain under intense investigation as they are technologically important in many areas ranging from microelectronics to medicine [1] , [2] , [3] , [4] , [5] , [6] , [7] , [8] , [9] , [10] , [11] , [12] , [13] , [14] , [15] , [16] . As a result, the continued discovery of new magnetic systems is of both fundamental scientific and practical importance. Confinement of magnetic species to the nanometre regime is known to enhance the magnetic properties [13] . The use of block copolymers (BCPs) to assemble nanoscopic elements with high density [17] , [18] (1 to 10 Terabits per square inch) is established, and attempts to exploit BCP templates to organize magnetic components has received considerable attention in the last two decades [19] , [20] . Although many strategies exist, they can be classified broadly into three different approaches that capitalize on the inherent nanoscopic order of the BCP. One approach involves using a highly oriented nanoporous template generated from BCPs for the electrochemical deposition of a magnetic material, like cobalt (Co), to produce nanorods on conducting substrates. Upon removing the minor component, Co was electrochemically deposited, resulting in small metal cylinders 14 nm in diameter with lengths of 500 nm and a coercivity ( H c ) of 800 Oe (Orsteds) [15] . A second approach selectively deposits the precursor of a magnetic material into one domain of the BCP followed by a reduction reaction to produce the magnetic material [21] , [22] , [23] , [24] . Using this strategy, Co nanoparticles were reported [21] with dimensions ranging from 10 to 288 nm and H c values between 20 and 360 Oe. It should be noted that CoFe 2 O 4 nanoparticles having diameters <5 nm were paramagnetic at room temperature [22] . Although this approach is perhaps simpler, it is difficult to exclusively confine the magnetic components to a single domain of the BCP. A third approach involves the incorporation of magnetic precursors directly into the chemical structure of the BCP. Pyrolysis has been typically used to convert the precursors into the corresponding magnetic material [25] , [26] , [27] . However, this results in a destruction of the nanostructured morphology. More recent efforts designed to conserve the BCP nanostructure did not lead to magnetic materials [28] . Here we report a method to encode BCPs with the chemical information required to self-assemble into nanostructures, which, upon a simple heat treatment, generates room temperature ferromagnetic materials (RTFMs) that retain the BCP morphology. The nanostructured morphologies (cylindrical, lamellar and inverted cylindrical) are shown to be essential, as the parent metal-containing homopolymer, lacking nanoconfinement, provides only superparamagnetic materials, even though it contains more Co. Further, the anisotropy of the one-dimensional cylindrical morphology is shown to give the highest H c , consistent with the strongest confinement. The method reported here demonstrates the role of BCP nanoconfinement on the fundamental magnetic properties of Co. It illustrates the ability to use BCP nanostructures to significantly alter the basic properties of the material. This approach is expected to produce more novel nanomaterials in the future. Polymer synthesis We synthesized a novel metal-containing monomer ( Fig. 1 ) and demonstrated its living ring-opening metathesis polymerization, as shown by both size exclusion chromatography and the dependence of number average molecular weight ( M n ) on the monomer to initiator ratio ( Supplementary Figs S1-S3 ). Five homopolymers with M n ranging from 20 to 100 kDa (degree of polymerization=41 to 208) and polydispersity index (PDI) of 1.1 were prepared. 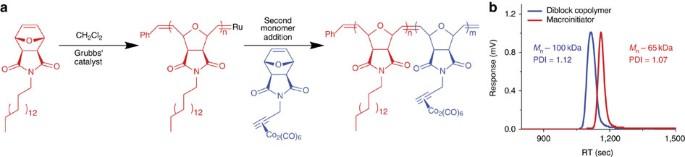Figure 1: Block copolymer synthesis. (a) Synthetic scheme of Co-containing BCPs prepared using Grubbs' third-generation catalyst. Using standard ring-opening metathesis polymerization conditions, the C16monomer was polymerized followed by BCP chain extension using the Co-containing monomer. (b) Two representative size exclusion chromatography curves highlighting the efficiency of BCP formation. The red curve is for the C16polymer chain, which was extended to form the diblock copolymer whose size exclusion chromatography is shown in blue. Figure 1: Block copolymer synthesis. ( a ) Synthetic scheme of Co-containing BCPs prepared using Grubbs' third-generation catalyst. Using standard ring-opening metathesis polymerization conditions, the C 16 monomer was polymerized followed by BCP chain extension using the Co-containing monomer. ( b ) Two representative size exclusion chromatography curves highlighting the efficiency of BCP formation. The red curve is for the C 16 polymer chain, which was extended to form the diblock copolymer whose size exclusion chromatography is shown in blue. Full size image The living polymerization of the metal-containing monomer is essential to produce a well-defined block topology. To enhance the second block's initiation efficiency, monomers having the same strained bicyclic structure were used ( Fig. 1 ). As shown in Figure 1 , BCPs were synthesized by the addition of the metal-containing monomer to a living block of an alkyl-chain-containing homopolymer. In this case, the first block had a M n of ∼ 65 kDa and the BCP had a total M n of ∼ 100 kDa. The fidelity and quantitative conversion of the polymerizations are shown by size exclusion chromatography. It should be noted that the reactions proceeded very rapidly; the total time for polymerization of the BCP was only ∼ 10 min. As the backbones of both blocks are the same, the alkyl chain length of the non-metal-containing block is important in driving microphase separation of the BCP. Three different monomers were prepared with alkyl chain lengths of 5, 9 and 16. From scanning force microscopy measurements, the C 16 -containing BCP showed the largest, most well-developed microdomains, followed by the C 9 and C 5 copolymers ( Supplementary Fig. S4 ). Consequently, only the C 16 -containing BCP was studied further. Block copolymer nanostructure Small-angle X-ray scattering (SAXS) and transmission electron microscopy (TEM) were used to characterize the BCP morphology before and after the heat treatment. SAXS showed two reflections occurring at scattering vectors of 1 and √3 times the first-order reflection, which is consistent with a cylindrical microdomain morphology ( Supplementary Fig. S5 ). 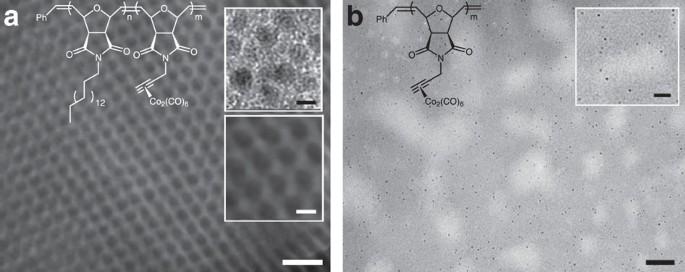Figure 2: Morphology of BCP and homopolymer. TEM images of an unstained, microtomed cross-section of a thermally annealed, Co-containing (a) BCP (scale bar, 100 nm) and (b) homopolymer (scale bar, 100 nm) showing the cylindrical microdomain morphology of the BCP and Co nanoparticles distributed randomly in the homopolymer (inset scale bar, 20 nm). Insets in (a) magnify the cylindrical domains (both white and black scale bars in insets are 20 nm) with the largest magnification and thinner microtomed section showing small metal nanoparticles inside the cylinders. A TEM image of a microtomed, unstained sample after heat treatment is shown in Figure 2a . The contrast arises from the presence of Co in the cylindrical microdomains. The TEM and SAXS results are consistent with ∼ 20 nm diameter cylindrical microdomains with a center-to-center distance of ∼ 40 nm. Figure 2: Morphology of BCP and homopolymer. TEM images of an unstained, microtomed cross-section of a thermally annealed, Co-containing ( a ) BCP (scale bar, 100 nm) and ( b ) homopolymer (scale bar, 100 nm) showing the cylindrical microdomain morphology of the BCP and Co nanoparticles distributed randomly in the homopolymer (inset scale bar, 20 nm). Insets in ( a ) magnify the cylindrical domains (both white and black scale bars in insets are 20 nm) with the largest magnification and thinner microtomed section showing small metal nanoparticles inside the cylinders. Full size image The thermal removal of the carbonyl ligands on dicobalt hexacarbonyl metal complexes is well known [29] , [30] , [31] , [32] , [33] , [34] . Thermal gravimetric analysis showed the loss of the carbonyl moieties occurred from ∼ 110 to 200 °C for the BCP at a heating rate of 10 °C min −1 ( Supplementary Figs S6 and S7 ). The weight loss indicated that 94% of the carbonyl ligands were removed. Similar results were obtained by heating the sample to 120 °C for 12 h. SAXS and TEM, before and after thermal treatment showed no significant changes in the morphology ( Supplementary Fig. S8 ). For the homopolymer, no distinct features were observed by TEM or SAXS before heating ( Supplementary Fig. S9 ). However, after thermal annealing, a random distribution of nanoparticles within the homopolymer matrix was observed ( Fig. 2b ). These Co particles, ∼ 5 nm in diameter, are too small to be inherently ferromagnetic at room temperature. Extensive TEM on ultrathin microtomed slices of the BCP showed similar particles within the cylindrical domains ( Fig. 2a inset). Magnetic property measurements Following thermal treatment, the BCPs were found to be ferromagnetic, whereas the homopolymers were paramagnetic in keeping with the smaller size of the nanoparticles randomly distributed in the homopolymer. Both the BCP and homopolymer were black, following thermal annealing, which is consistent with the formation of nanoscopic Co-based particles. 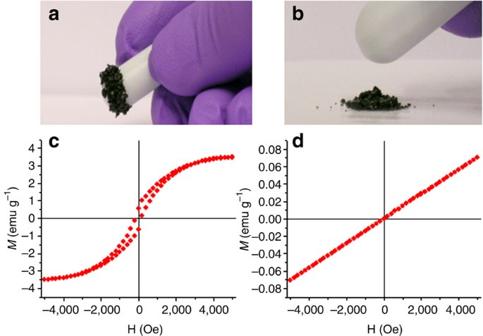Figure 3: Magnetic characterization of the BCP and homopolymer. The room temperature response of the thermally annealed (a) BCP and (b) homopolymer to a permanent magnet along with superconducting quantum interference device magnetometer measurements to quantify their magnetic properties. The (c) BCP is ferromagnetic at room temperature, whereas the (d) homopolymer is paramagnetic. However, the responses of the BCP and homopolymer to a permanent magnet are markedly different, as shown in Figure 3a,b . This image shows that the BCP is strongly attracted to the magnet, whereas the homopolymer is unresponsive ( Supplementary Movie 1 ). A superconducting quantum interference device magnetometer was used to characterize the magnetic properties of these two materials. The homopolymer ( Fig. 3d ) is superparamagnetic with a H c of zero, which is consistent with previous reports on Co nanoparticles with diameters of ∼ 5 nm or less [14] , [35] . However, after annealing, the BCPs showed ferromagnetic behaviour at room temperature ( Fig. 3c ). The saturation magnetization, remanent magnetization and H c were found to be 3.5 emu g −1 , 0.61 emu g −1 and 200 Oe, respectively. The difference in the behaviour of the BCP and homopolymer is even more notable when the higher concentration of Co in the homopolymer (26 wt%) is compared with the BCP (14 wt%). Field-cooling experiments confirmed that the BCP is ferromagnetic and that homopolymer is paramagnetic ( Supplementary Figs S10 and S11 ). Figure 3: Magnetic characterization of the BCP and homopolymer. The room temperature response of the thermally annealed ( a ) BCP and ( b ) homopolymer to a permanent magnet along with superconducting quantum interference device magnetometer measurements to quantify their magnetic properties. The ( c ) BCP is ferromagnetic at room temperature, whereas the ( d ) homopolymer is paramagnetic. Full size image Cobalt structure Crystalline Co nanoparticles, having an average diameter of 5 nm, were grown by known solution methods [36] , and mixed with the C 16 homopolymer so that the total Co content was 10 wt%, lower than the Co content of the BCP or homopolymer samples. 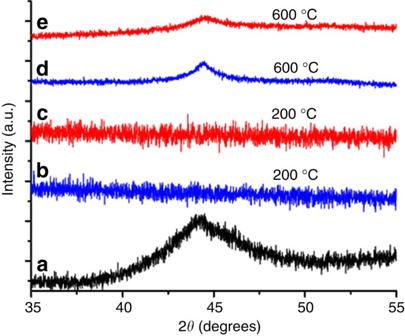Figure 4: Characterization of the Co particle structure. Wide-angle X-ray diffraction profiles of (a) a 10 wt% blend of solution prepared crystalline Co nanoparticles in the C16-containing homopolymer, the 200 °C-treated (b) BCP and (c) homopolymer (identical to those shown inFig. 3), and the 600 °C-pyrolyzed samples of the (d) BCP and (e) homopolymer, which removes all the organic ligands and allows the Co present to crystallize. The wide-angle X-ray diffraction of this mixture is shown in Figure 4a where a clear signal was observed for the Co nanocrystals. The wide-angle X-ray diffraction profiles in Figure 4b,c were collected from the Co-containing BCP and homopolymer samples prepared identically to those described in Figure 3 . No reflection was observed between 40–55° (2 θ ), as would be expected for Co nanocrystals. From the results in Figure 4a , the absence of reflections cannot be attributed to a size or concentration effect. Figure 4d,e show the diffraction profiles of the BCP and homopolymer samples after pyrolysis at 600 °C. Upon removal of the organic material by pyrolysis, the Co present in the sample is able to crystallize, confirming that the presence of the organic acetylene ligands were responsible for preventing crystallization. Figure 4: Characterization of the Co particle structure. Wide-angle X-ray diffraction profiles of ( a ) a 10 wt% blend of solution prepared crystalline Co nanoparticles in the C 16 -containing homopolymer, the 200 °C-treated ( b ) BCP and ( c ) homopolymer (identical to those shown in Fig. 3 ), and the 600 °C-pyrolyzed samples of the ( d ) BCP and ( e ) homopolymer, which removes all the organic ligands and allows the Co present to crystallize. Full size image Selected area electron diffraction and high-resolution TEM studies on the Co-containing BCP and homopolymer samples showed no evidence of Co crystals in samples heated to 200 °C. Taken together, these results suggest that the Co in the BCP and homopolymer is not crystalline; however, the BCP is clearly a RTFM. Amorphous magnetic materials containing Co are known [37] , [38] , [39] , [40] . Near-edge X-ray absorption fine structure spectroscopy of the BCP and homopolymer before and after heat treatment confirmed the presence of only Co metal species within the polymers ( Supplementary Fig. S12 ). A single, absorption edge was observed at 781 eV, consistent with small Co metal nanoparticles [41] . The origin of the RTFM properties arises from the nanostructured confinement of Co within the one-dimensional cylinders of the BCP morphology. This is supported by the fact that small nanoparticles ( ∼ 5 nm), too small to be inherently ferromagnetic at room temperature, are present in both the BCP and unstructured homopolymer. To further support this hypothesis, a series of BCPs were prepared in which the BCP morphology was varied between the cylindrical, lamellar, and inverted cylindrical phases ( Supplementary Table S1 ). 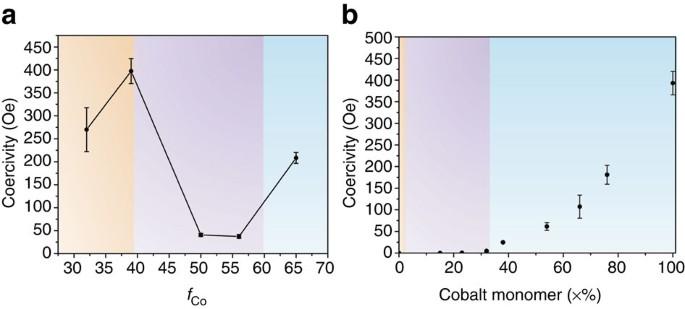Figure 5: Effect of confinement on magnetic properties. (a) Effect of confinement in the diblock copolymer morphologies on their coercivity. The shaded regions correspond to: (orange)—cylindrical morphology; (purple)—lamellar morphology; (blue)—inverted cylindrical morphology. (b) Effect of dilution of cobalt density within cylindrical phase by varying the ratio of the monomers containing cobalt and ferrocene in the metal block of diblock copolymer. The shaded regions correspond to: (orange)—diamagnetic; (purple)—paramagnetic; (blue)—ferromagnetic behaviour. Figure 5a shows the H c as a function of BCP morphology following the heat treatment. First, it should be noted that all BCP morphologies provide RTFM materials. In other words, nanostructuring leads to RTFM properties in all cases in contrast to the unstructured homopolymer, which is never ferromagnetic. Second, and consistent with expectations, the cylindrical BCP, which is the most strongly confined, has the largest H c . Similarly, the inverted cylindrical phase, often considered as a three-dimensional phase due to the interconnectivity (or percolation) of the matrix block, shows the second highest H c . This is due to the confinement between cylinders, which is overall weaker than the cylindrical phase but stronger than the lamellar morphology. Therefore, it becomes clear that confinement within the 1-D cylindrical phase imparts an additional interaction among the Co particles leading to increased magnetic coupling among them and thus RTFM properties. Figure 5: Effect of confinement on magnetic properties. ( a ) Effect of confinement in the diblock copolymer morphologies on their coercivity. The shaded regions correspond to: (orange)—cylindrical morphology; (purple)—lamellar morphology; (blue)—inverted cylindrical morphology. ( b ) Effect of dilution of cobalt density within cylindrical phase by varying the ratio of the monomers containing cobalt and ferrocene in the metal block of diblock copolymer. The shaded regions correspond to: (orange)—diamagnetic; (purple)—paramagnetic; (blue)—ferromagnetic behaviour. Full size image This increased magnetic coupling due to confinement was evaluated by effectively 'diluting' the Co density within the cylindrical phase. A new BCP ( Supplementary Fig. S13 ) was designed in which the metal block of the BCP contained the original Co monomer as well as a new metal-ion-containing monomer. This new monomer, based on ferrocene, was chosen, as it is inert to the annealing conditions but still imparts phase-separation properties for the BCP ( Supplementary Figs S13 and S14 ). Thus, it served simply to reduce the effective Co density within the BCP. It was proposed that this reduced Co density would lead to reduced magnetic coupling among the formed Co nanoparticles. Keeping the cylindrical phase constant (total BCP MW and block ratios), the ratio of Fe to Co monomer was systemically varied from 0 to 100% Co. Figure 5b shows that below a critical threshold of 30 mol% Co; essentially no H c was measured. However, as the Co percentage increased, the corresponding H c ( Supplementary Fig. S15 ) also increased, reaching a maximum of 393 Oe at 100% Co monomer. These results demonstrate clearly that Co density within the cylinder directly affects the RTFM properties of the materials and again illustrates the importance of nanostructured confinement. A direct comparison with other systems reported in the literature is difficult, as magnetic properties are known to depend on the size, shape and density of the magnetic components [13] . However, the BCP's H c is 20–40 times larger than that of a continuous Co film ( H c =10 Oe) [15] and comparable to the H c (186–209 Oe) reported for hexagonally packed cylinders (20 nm diameter) grown in alumina membranes [42] . Cobalt nanoparticles with dimensions similar to the cylinder diameter of the BCP reported H c values of 68 Oe [21] . The process outlined here leads to environmentally stable magnetic materials over extended time periods. When the magnetization of the BCP was measured for the exact same sample 4 months later, identical moment versus field curves were generated. Noting that the magnetic behaviour observed for this BCP is seen in other Co-containing BCPs and not the corresponding homopolymers, the approach appears to be general. Our results demonstrate a route to influencing the materials' magnetic properties by nanostructuring. It is the strong confinement, particularly of the cylindrical domain, that is responsible for the observed room temperature ferromagnetic properties. This approach is extremely simple in comparison with previously reported systems, as it only involves film casting followed by a relatively low-thermal treatment. The ability to use BCP nanoconfinement to profoundly alter the foundational properties of a material holds significant promise for future nanomaterials. Block copolymer synthesis Known amounts of monomers were added into two separate Schlenk flasks under an atmosphere of nitrogen, and dissolved in anhydrous CH 2 Cl 2 (1 ml per 100 mg of monomer). A desired amount of third-generation Grubbs' catalyst was added into another Schlenk flask, flushed with nitrogen and dissolved in a minimum amount of anhydrous CH 2 Cl 2 . All three solutions were degassed by three freeze–pump–thaw cycles. First, monomer was transferred to the flask containing the catalyst via a cannula. The reaction mixture was stirred vigorously for 5 min, after which an aliquot was taken for gel permeation chromatography analysis, and the second monomer was transferred to the flask via a cannula. The polymerization was allowed to continue for another 5 min, and then quenched with 0.2 ml of ethyl vinyl ether. An aliquot was taken for gel permeation chromatography analysis, and the remaining product was precipitated from methanol. TEM and SAXS measurements Samples for TEM were prepared by drop-casting a 10 wt% toluene solution into a Teflon mould, the sample was then solvent annealed in benzene for 2 weeks, embedded in an epoxy resin and cured at 60 °C for 24 h. Ultrathin sections were then cut with a diamond knife using a Leica Ultracut microtome. TEM analysis was conducted on a JEOL 100CX TEM operating at an accelerating voltage of 100 kV. For samples studied after annealing, the samples were heated to 200 °C after solvent annealing but before epoxy treatment. Small-angle x-ray scattering samples were prepared by drop-casting a 10 wt% toluene solution into a Teflon mould, the sample was then solvent annealed in benzene for 2 weeks before sandwiching between Kapton films. The calculated center-to-center d-spacing of microdomains was found to be 40 nm. Magnetic measurements Polymer samples were dissolved in toluene to form 10 wt% solutions. These solutions were evaporated under a nitrogen stream and then thermally annealed in a tube-furnace under vacuum at 200 °C for 6 h. The films were powdered and filled into a gelatin capsule, inserted into a straw and placed into the Quantum Design MPMS superconducting quantum interface device magnetometer. The magnetic characterization was performed at room temperature by varying the field from −10,000 to 10,000 Oe. The H c , saturation magnetization and remanent magnetization were determined. How to cite this article: AL-Badri, Z. M. et al . Room temperature magnetic materials from nanostructured diblock copolymers. Nat. Commun. 2:482 doi: 10.1038/ncomms1485 (2011).